Soft X-ray spectromicroscopy using ptychography with randomly phased illumination Ptychography is rapidly developing into an important tool in X-ray microscopy. The technique involves successively illuminating overlapping regions of a specimen with a localized probe and recording the resulting diffraction patterns. A key requirement is that the illuminated areas overlap substantially, so that iterative algorithms [1] , [2] , [3] can successfully reconstruct an image of the specimen, retrieving the amplitude and phase of both the complex sample transmission function and the illuminating probe. At X-ray wavelengths, ptychography has been used to characterize the focusing properties of X-ray optics [4] , [5] , [6] , to image interconnects within microchips [7] and to image yeast cells [8] . X-ray ptychography has recently been demonstrated using soft X-rays [9] , [10] , and has been used with polarized illumination to generate dichroic image contrast from magnetic thin films [11] . It can also be combined with tomography to produce three-dimensional reconstructions [12] , [13] , [14] . Despite these successes, ptychographic imaging suffers from the same recurring problem as coherent diffraction imaging, in that the diffraction patterns generally have an extremely large dynamic range, with a zero-order component orders of magnitude more intense than the scattered signal. As a result, multiple exposures may be needed to allow accurate recording of the full dynamic range of the diffraction pattern or a beamstop may be introduced to block the zero-order component. However, as some ptychographic algorithms do not require a priori knowledge of the form of the illuminating probe, but can extract this information from the recorded data sets, it is possible to consider enhancing the phase diversity of the probe to reduce the dynamic range of the recorded diffraction data and improve the quality of the reconstructed image [15] , [16] . This approach is conceptually similar to the use of coded-aperture imaging at visible [17] and X-ray wavelengths [18] , except that the ptychographic approach does not require a priori knowledge of the coded apertures to achieve successful image reconstructions. At visible-light wavelengths, a diffuser was used to randomize the phase structure of the ptychographic probe [15] . Here we demonstrate the method in the soft X-ray regime, reducing the dynamic range of the diffraction patterns by an order of magnitude. In this case, the phase diversity of the probe was enhanced by introducing into the beam path a pseudo-random array of ~40 nm diameter holes in a 140-nm thick tungsten film. We show that despite the complexity of the probe wavefront, samples with relatively small X-ray-scattering cross-sections can be imaged successfully. A recent mathematical analysis has shown that randomly phased illumination can also help standard phasing algorithms converge more rapidly to a reliable solution [19] . We employ our novel experimental geometry to generate a series of ptychographic reconstructions at X-ray energies around the L absorption edge of iron, demonstrating chemical sensitivity without the need for optical refocusing. The amplitude and phase of the complex sample transmittance are recovered simultaneously by the ptychographic reconstructions, in perfect registration and at the same spatial resolution, allowing a major enhancement of the information normally available from near-edge X-ray spectromicroscopy. In particular, our results show that the phase signal can provide a more sensitive indication of changes in the local chemical environment. Description of the experiment Experiments were carried out using the TwinMic X-ray microscope at the Elettra facility [20] . TwinMic has the unique capability to operate as both a transmission X-ray microscope (TXM) and as a scanning TXM (STXM). A hybrid mode involving both aspects was used for our ptychography experiments, as shown schematically in Fig. 1 . 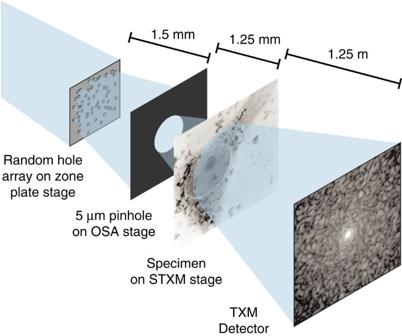Figure 1: Schematic representation of the modified experimental setup on the TwinMic beamline. A monochromatic X-ray beam illuminates an array of randomly positioned pinholes (~40 nm diameter) that replaces the zone plate normally used during STXM operation of the TwinMic instrument. The pinholes act to diffuse the illumination and part of this diffuse beam is selected by a beam-defining pinhole that occupies the order-selecting aperture (OSA) stage used in STXM mode. The specimen sits on the standard STXM stage and is scanned across the beam in small rasters. The CCD normally used for imaging in TXM mode is used to record the diffraction pattern produced by the sample for every position in the raster scan. Figure 1: Schematic representation of the modified experimental setup on the TwinMic beamline. A monochromatic X-ray beam illuminates an array of randomly positioned pinholes (~40 nm diameter) that replaces the zone plate normally used during STXM operation of the TwinMic instrument. The pinholes act to diffuse the illumination and part of this diffuse beam is selected by a beam-defining pinhole that occupies the order-selecting aperture (OSA) stage used in STXM mode. The specimen sits on the standard STXM stage and is scanned across the beam in small rasters. The CCD normally used for imaging in TXM mode is used to record the diffraction pattern produced by the sample for every position in the raster scan. Full size image To assess the effectiveness of the random hole array in reducing the dynamic range of the diffraction data, diffraction patterns were recorded from the 5-μm probe-defining pinhole alone, and when the hole array was in position upstream of the 5-μm pinhole. Three exposures were recorded in each case: at 1, 0.5 and 0.1 s for the pinhole alone, and 10, 5 and 1 s for the combination of the pinhole and the random hole array, which absorbed approximately 70% of the incident beam at energies around 700 eV. These exposures were combined to produce the results shown in Fig. 2 , from which it is clear that the random hole array has significantly increased the fraction of the signal distributed across the detector plane, by about an order of magnitude. 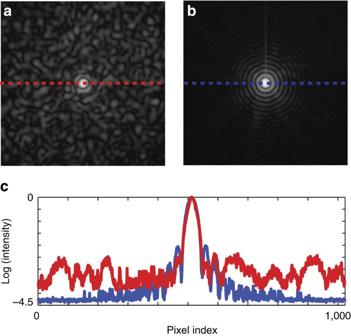Figure 2: Diffraction patterns recorded in the absence of a sample. The diffraction patterns inaandbwere obtained by the combination of three different exposures and are shown with logarithmic scaling of the intensity. (a) The pattern obtained with the random-hole array in place upstream of the 5-μm pinhole using exposures of 10, 5 and 1 s. (b) The pattern obtained with only the 5-μm pinhole using exposures of 1, 0.5 and 0.1 s. (c) Line plots of the intensity along the dashed lines inaandb. Figure 2a retains a relatively intense central spot, so that a significant further reduction in dynamic range could be achieved by improving our method of randomizing the phase in the pinhole plane. Figure 2: Diffraction patterns recorded in the absence of a sample. The diffraction patterns in a and b were obtained by the combination of three different exposures and are shown with logarithmic scaling of the intensity. ( a ) The pattern obtained with the random-hole array in place upstream of the 5-μm pinhole using exposures of 10, 5 and 1 s. ( b ) The pattern obtained with only the 5-μm pinhole using exposures of 1, 0.5 and 0.1 s. ( c ) Line plots of the intensity along the dashed lines in a and b . 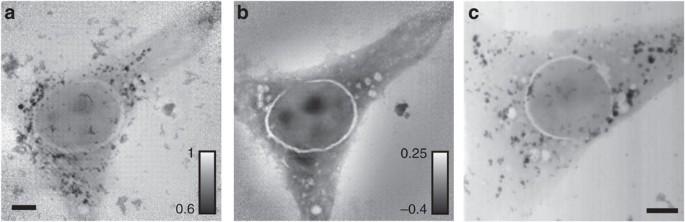Figure 3: Reconstructed modulus and phase images of a mouse Balb/3T3 fibroblast cell. The data foraandbwere recorded at an X-ray energy of 708.8 eV. The modulus scale is in arbitrary units and the phase scale in radians. (a) Modulus image, where the clusters of CoFe2O4nanoparticles appear as small dark spots. (b) Phase image, where the nanoparticle clusters have much lower contrast. (c) A conventional STXM absorption image of a similar mouse fibroblast cell taken at 707 eV with an X-ray probe size ~120 nm. Scale bar, 5 μm (inaandc). Full size image Figure 3 shows the reconstructed modulus and phase of the specimen transmission function from a Balb/3T3 mouse fibroblast cell that had been doped with cobalt ferrite (CoFe 2 O 4 ) nanoparticles [21] . The set of diffraction patterns used for this reconstruction was collected at a beam energy of 708.8 eV from a regular grid of 27 × 27 specimen positions, with a grid spacing of 1 μm. Clusters of CoFe 2 O 4 particles appear as small dark spots in the modulus image, concentrated mainly in the perinuclear region, but are not visible in the phase reconstruction. This is consistent with the theoretical values tabulated by Chantler [22] , [23] for the complex atomic X-ray-scattering factor at the iron L edge, which shows that the real part of the complex refractive index will have its minimum absolute value at around 708 eV, while this energy marks the onset of the absorption edge. Figure 3: Reconstructed modulus and phase images of a mouse Balb/3T3 fibroblast cell. The data for a and b were recorded at an X-ray energy of 708.8 eV. The modulus scale is in arbitrary units and the phase scale in radians. ( a ) Modulus image, where the clusters of CoFe 2 O 4 nanoparticles appear as small dark spots. ( b ) Phase image, where the nanoparticle clusters have much lower contrast. ( c ) A conventional STXM absorption image of a similar mouse fibroblast cell taken at 707 eV with an X-ray probe size ~120 nm. Scale bar, 5 μm (in a and c ). Full size image The incident X-ray probe is recovered simultaneously by the extended ptychographical iterative engine (ePIE) reconstruction [3] and is shown in Fig. 4a , where brightness represents the amplitude and hue represents the phase. Propagating the probe upstream to the plane of the pinhole produces Fig. 4b : the shape of the pinhole is well defined, with a diameter ~5 μm, and the structure of the wavefront within it demonstrates the effectiveness of the random hole array as a diffusing mask. 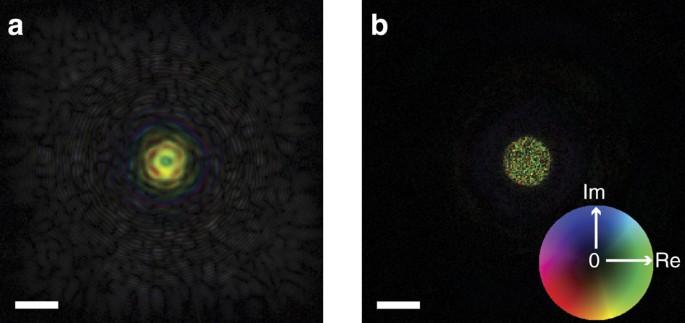Figure 4: Reconstructed probe wavefront. The real and imaginary parts of the reconstructed wavefront are shown using a colorwheel scale. (a) Reconstruction at the sample plane. (b) The wavefront after propagation upstream to the pinhole plane. Scale bar, 5 μm. Figure 4: Reconstructed probe wavefront. The real and imaginary parts of the reconstructed wavefront are shown using a colorwheel scale. ( a ) Reconstruction at the sample plane. ( b ) The wavefront after propagation upstream to the pinhole plane. Scale bar, 5 μm. Full size image One issue with our method is the difficulty of sufficiently localizing the probe at the plane of the sample, a problem also noted by Giewekemeyer et al . [9] . This was exacerbated in our case by the requirement to bin the diffraction data (see Methods section). Consequently a small degree of aliasing at the extremities of the probe reconstruction did produce some low intensity noise beyond the aperture of the pinhole that is too dim to be seen in Fig. 4b . The ptychographic reconstructions in Fig. 3a have an estimated resolution 250 nm, which is significantly smaller than the probe size on the sample, and have levels of image detail and contrast that are directly comparable to the conventional STXM absorption image shown in Fig. 3c . This image was acquired using zone-plate optics to produce an X-ray probe size ~120 nm. 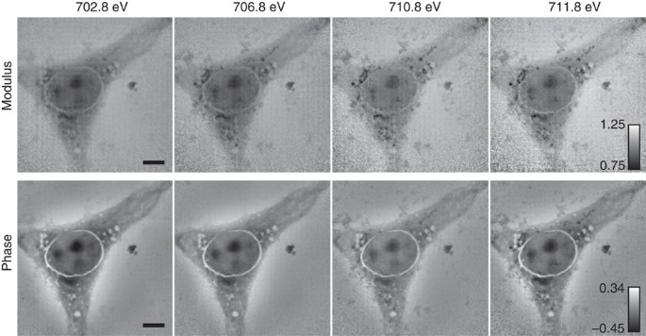Figure 5: Reconstructed modulus and phase images of a Balb/3T3 mouse fibroblast. The data were collected at X-ray beam energies across the iron L edge, showing the variation in contrast of the CoFe2O4nanoparticles as a function of energy. Scale bar, 5 μm. Imaging at energies around the iron L edge Figure 5 shows ptychographic reconstructions from data collected at four other energies around the Fe L 3 edge. In these scans, the raster size was 18 × 18 and the grid spacing was 1.5 μm. The figure shows that the changes in image contrast from the CoFe 2 O 4 particles are significantly different for the modulus and phase signals. Assuming the sample is sufficiently thin to be modelled by a multiplicative complex transmission function , where the complex refractive index n ( r )=1− δ ( r )+ iβ ( r ), t ( r ) is the local thickness of the sample and λ is the wavelength of the illumination, then the optical thickness ( n ( r )−1) t ( r ) can be found directly from the ptychographic reconstructions. In particular, the phase image contrast is proportional to −2 π δ t / λ , while the natural log of the modulus image gives −2 πβt / λ . In addition, the optical thickness can be separated into two components: one associated with the organic matter of the cell, and the other associated with the CoFe 2 O 4 nanoparticles. The first of these components will be almost constant for small energy changes around the Fe L edge, so the difference between two phase images at nearby energies yields a signal that relates directly to the optical thickness of the CoFe 2 O 4 nanoparticles. The same is true for the difference between two log e (modulus) images taken at nearby energies. Figure 5: Reconstructed modulus and phase images of a Balb/3T3 mouse fibroblast. The data were collected at X-ray beam energies across the iron L edge, showing the variation in contrast of the CoFe 2 O 4 nanoparticles as a function of energy. Scale bar, 5 μm. Full size image Regions of interest (RoI) were defined by subtracting two phase images at nearby energies to produce a binary mask that could be applied to all the phase and log e (modulus) images, allowing statistical data to be obtained for 66 RoI where the contrast was changing as a function of energy. The results of this analysis are plotted in Fig. 6 , which shows the variation of log e (modulus) and phase with energy for RoI that have been separated into five different classes. The values of −2 πβt / λ and −2 πδt / λ for CoFe 2 O 4 calculated using Chantler’s compilation of atomic scattering factors [22] , [23] are plotted on the same graph, using a nominal CoFe 2 O 4 thickness of t =90 nm to ensure that the vertical scaling of the calculated data approximately matches the experimentally observed variations in the signals. To make comparison easier, a vertical offset has been added to our measurements of the class-average values for the RoI, so that they lie on the curves of Chantler’s data at the lowest energy (697.8 eV). To our knowledge, there are no published measurements of the phase variation across the Fe L edge for CoFe 2 O 4 , but measurements of the X-ray absorption spectrum and the X-ray magnetic circular dichroism signal have been made by Pattrick et al . [24] and on CoFe 2 O 4 nanoparticles by Coker et al . [25] , who kindly provided their total electron yield (TEY) measurements of absorption across the Fe L edge (V. S. Coker, personal communication). Although it is difficult to make a direct comparison between TEY measurements and thin-film X-ray transmission data, a logarithmically scaled version of these TEY data is also plotted on Fig. 6 to provide a comparison with the log e (modulus) data. The TEY data were also used to provide a more accurate energy calibration of the data available from the monochromator on the TwinMic beamline at Elettra. Average values for each class of the RoI are plotted in a separate colour in Fig. 6 , and dots with the same colours identify the locations of the RoI on the inset phase image. 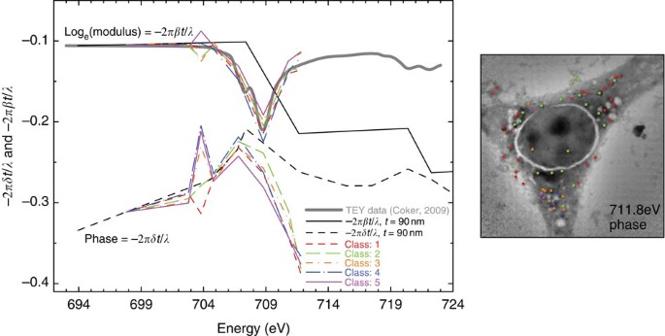Figure 6: Plot of the loge(modulus) and phase image signals measured from the CoFe2O4nanoparticles. The locations of the nanoparticle clusters are highlighted by coloured dots in the inset image (phase image at 711.8 eV). The curves show that five different classes of behaviour as a function of X-ray energy were identified. For comparison, a scaled plot of the TEY signal from similar particles25is overlaid on the loge(modulus) plots, along with curves calculated for a 90-nm thick film of CoFe2O4derived from the semi-empirical tabulation by Chantler22,23. Figure 6: Plot of the log e (modulus) and phase image signals measured from the CoFe 2 O 4 nanoparticles. The locations of the nanoparticle clusters are highlighted by coloured dots in the inset image (phase image at 711.8 eV). The curves show that five different classes of behaviour as a function of X-ray energy were identified. For comparison, a scaled plot of the TEY signal from similar particles [25] is overlaid on the log e (modulus) plots, along with curves calculated for a 90-nm thick film of CoFe 2 O 4 derived from the semi-empirical tabulation by Chantler [22] , [23] . Full size image We have shown how one of the major practical difficulties of X-ray ptychography, the extremely large dynamic range of the diffraction patterns, can be alleviated at soft X-ray energies by introducing a suitable diffusing structure into the probe-forming optics. Our method is equally applicable at hard X-ray energies, and indeed the diffusing structure is easier to realize at these shorter wavelengths. We have also shown that the added complexity of the probe does not adversely affect the robustness and reliability of the reconstruction algorithm and that quantitative reconstructions of weakly scattering samples are possible using this experimental geometry. One difficulty we have encountered is that of suitably localizing the structured probe at the sample plane. The combination of a diffusing structure with a focusing optic could alleviate this issue. Two previous studies have combined ptychography with beam-energy changes to realize chemically sensitive imaging. Beckers et al . [10] used the absorption and phase changes at five energies across the oxygen K edge to distinguish between 2-μm diameter spheres of polymethyl methacrylate and silicon dioxide. Takahashi et al . [26] also made measurements of the phase signal at two energies below the Au M edge (around 11.9 keV) to study the distribution of Au in Au/Ag nanoparticles. In our case, ptychographic data were collected at eight energies between 697.8 and 711.8 eV, and we have been able to show that both the modulus and the phase signals are sensitive to the chemical environment of the Fe atoms present in the CoFe 2 O 4 nanoparticles. The general shape of the measured log e (modulus) data matches well the TEY data taken from similar nanoparticles, while it is clear that the phase variations across the edge can give stronger and clearer features than the modulus data provided. It is also reassuring to note that the phase variation across the edge broadly follows the tabulated data from Chantler [22] , [23] , with the notable exception that the tabulated data do not show the very prominent pre-edge peak or dip that is measured experimentally around 704 eV. From the shapes of the log e (modulus) and phase variations across the edge, even on the relatively sparse set of data presented here, it is possible to see that the iron exists in a number of different chemical states. The X-ray magnetic circular dichroism measurements by Coker et al . [25] suggested that at least three forms of iron were present: octahedrally coordinated Fe 2+ and Fe 3+ and tetrahedrally coordinated Fe 3+ . Calculations of the 2 p absorption spectra for iron with these symmetries indicate that the observed spectra will depend on 2 p– 3 d and 3 d– 3 d Coulomb and exchange interactions, 2 p and 3 d spin-orbit interactions and the crystal field acting on the 3 d states [27] . The sparse nature of the spectral data in Fig. 6 does not allow a more detailed analysis of the components present in the different RoI classes. However, the distribution of the coloured dots in the inset image does show that particles in RoI class 2 lie predominantly in the perinuclear region, whereas those in class 1 lie further from the nucleus. The other three classes occur much less frequently, and almost all of them are found close together on the arm of the fibroblast in the lower part of the image field. It is not possible to determine from these limited data whether the changes in the chemical environment of the iron result directly from biodegradation within the cellular environment. The ptychographic approach to imaging offers some important advantages for high-resolution X-ray spectromicroscopy. It provides modulus and phase reconstructions with a spatial resolution which is comparable to that achieved when the TwinMic microscope is operated as a conventional STXM, while the use of a relatively large probe on the sample allows a usefully large area to be covered in a raster of modest size, with no refocusing required when the incident X-ray energy was changed. At present, a rate-limiting step for our measurements is the time needed to readout the CCD (charge-coupled device) detector, but faster CCD systems are now available and it is reasonable to assume that much faster scans will be possible in future with an optimized system. We have also shown that near-edge measurements of the phase signal provide new information that complements and supplements that available from near-edge X-ray absorption fine structure (NEXAFS) measurements. NEXAFS imaging in the X-ray microscope has become a vital tool for the study and chemical characterization of nanoscale materials [28] , [29] , but hitherto the use of near-edge phase information has mostly relied on resonant soft X-ray reflectivity measurements [30] . Another promising approach involves the combination of multiple-wavelength anomalous diffraction with soft X-ray holography [31] , but this method requires a priori knowledge of the optical constants as a function of wavelength to provide high-resolution reconstructions that are sensitive to the elemental, chemical and magnetic state at the nanoscale. At present, there is a dearth of detailed experimental and theoretical data on the fine structure of phase variations near to absorption edges, and we believe that the ability of X-ray ptychography to provide direct, quantitative phase information in perfect registration with conventional NEXAFS data will open up a rich new branch of X-ray spectromicroscopy. Experimental method The soft X-ray diffuser consisted of a pseudo-random array of ~40 nm diameter holes in a 140-nm thick tungsten film in the beam path. The holes covered about a quarter of a 95 × 95 μm 2 field in the tungsten film, with hole positions determined by the Mersenne Twister algorithm [32] to avoid systematic correlations. Random hole patterns were supplied to our specification by Zoneplates Ltd, London, UK. The holes in the film acted as secondary sources with randomized phases, giving a diffuse, highly speckled beam downstream of the hole array. A 5-μm pinhole placed in this beam produced a localized probe in the sample plane. The sample was scanned in small rasters transverse to the beam direction, with step sizes ~1 μm, allowing a series of diffraction patterns to be recorded from overlapping areas using the X-ray sensitive CCD normally used for imaging in the TXM mode. The TXM camera was capable of outputting 16-bit images each of 1340 × 1300 pixels on a 20-μm pitch. It was operated in accumulation mode, capturing 8 frames, each of 0.5 s dwell time, from each position in the raster. Memory limitations required that the recorded data be binned by a factor of 4, and the resulting 335 × 325 pixel CCD frames were then cropped to 256 × 256 pixels. After each raster scan, a darkfield measurement was taken with the same camera settings and the beamline shutter closed, and this was subtracted from each diffraction pattern in the data set. No further efforts to mitigate noise in the data were undertaken. Reconstruction procedure Images were reconstructed using the ePIE method described by Maiden and Rodenburg [3] . The signal within a central disc of diameter 10 pixels was distorted by saturation in the binned diffraction patterns, but by allowing the signal to ‘float’ in this region (so that the diffraction constraint was not applied within this area during the course of the reconstruction), the ePIE method successfully reintroduced a smooth central peak into the diffraction data [33] . It is better to use an irregular grid of illumination positions for ptychography to avoid periodic, ill-constrained features in the reconstruction. However, the STXM stage-control software was designed to perform only regular raster scans, so small random fluctuations in the specimen positions (within ±0.5 pixels) were introduced and varied during the reconstruction, thus breaking the regularity of the actual positions at the expense of a small loss in the attainable resolution. Averaging over the final 25 ePIE iterations further reduced noise in the reconstructed image. Because each ePIE iteration involves updating the current specimen estimate once for each of the N recorded diffraction patterns, this averaging was taken over the final 25 N specimen estimates. The phase reconstructions are consistent in quality across the absorption edge and show very little noise at any energy. Although the modulus images are somewhat noisier, and they degrade slightly at energies below the absorption edge, the ePIE does not diverge. Image analysis Reconstructions at eight different energies were all re-sampled to the same pixel size, and the phase reconstructions packed into a three-dimensional stack that was aligned using the Multistackreg plug-in for ImageJ [34] , [35] . The same transformations were then applied to a similar stack of log e (modulus) images to produce two mutually aligned sets of data. The ptychographic image data were reconstructed with pixel sizes ~80 nm, which is almost two orders of magnitude smaller than the size of the illumination spot on the sample plane. As the features in the fibroblast cells are not of well-defined sizes and shapes, it is hard to get a precise determination of the spatial resolution in the reconstructions, but an estimate can be made by considering the signal profile across the boundary of the cell nucleus that appears as a bright ring in the phase reconstructions. The Straighten plug-in for ImageJ [34] was used to select arcs about 40 pixels wide that straddled part of the nuclear perimeter, the arcs were straightened using the method described in Kocsis et al . [36] and then line profiles perpendicular to the arc were used to estimate the sharpness of the edge. The separation of 10–90% contours suggested that a spatial resolution ~250 nm was achieved in the reconstructions, but in practice this should be considered an upper-limit (worst-case) estimate, because the cell boundary may not be sharply defined, and the process of arc selection, interpolation and alignment may well result in some broadening of the edge. How to cite this article: Maiden, A.M. et al . Soft X-ray spectromicroscopy using ptychography with randomly phased illumination. Nat. Commun. 4:1669 doi: 10.1038/ncomms2640 (2013).